Genetic deficiency of the mitochondrial protein PGAM5 causes a Parkinson’s-like movement disorder Mitophagy is a specialized form of autophagy that selectively disposes of dysfunctional mitochondria. Delineating the molecular regulation of mitophagy is of great importance because defects in this process lead to a variety of mitochondrial diseases. Here we report that mice deficient for the mitochondrial protein, phosphoglycerate mutase family member 5 (PGAM5), displayed a Parkinson’s-like movement phenotype. We determined biochemically that PGAM5 is required for the stabilization of the mitophagy-inducing protein PINK1 on damaged mitochondria. Loss of PGAM5 disables PINK1-mediated mitophagy in vitro and leads to dopaminergic neurodegeneration and mild dopamine loss in vivo . Our data indicate that PGAM5 is a regulator of mitophagy essential for mitochondrial turnover and serves a cytoprotective function in dopaminergic neurons in vivo . Moreover, PGAM5 may provide a molecular link to study mitochondrial homeostasis and the pathogenesis of a movement disorder similar to Parkinson’s disease. Mitochondria have a primary physiological role in producing ATP as an energy source, but also regulate cell survival [1] , [2] . In response to cellular stress, dysfunctional mitochondria produce ROS and other pro-death mediators to initiate cell death programs, such as apoptosis, necroptosis, parthanatos or autophagic cell death [1] , [2] , [3] , [4] , [5] . Mitophagy, a selective form of autophagy, can target dysfunctional mitochondria for lysosomal degradation and protect cells from oxidative damage [6] . Several regulators of mitophagy, including PINK1, Nix (BNIP3L) and parkin have been identified [6] , [7] , [8] , [9] . Mutations or deletions of these genes have been associated with abnormal mitophagy. Abnormal mitophagy has been observed in a variety of diseases, including ischaemic injury and neurodegenerative disease [6] , [7] , [8] , [9] . Hence, understanding the detailed mechanism of mitophagy remains an important goal for improving the diagnosis and treatment of diseases involving mitochondria. Parkinson’s disease is the second most common neurodegenerative disease and is characterized by the selective loss of dopaminergic neurons [9] , [10] , [11] . Although the cause of death of dopamine (DA)-secreting neurons is still debated, oxidative stress originating from mitochondria and mitophagy defects have been proposed to contribute to disease pathogenesis [12] , [13] . Two autosomal recessive Parkinson’s disease genes, PINK1 (PTEN-induced putative kinase 1) and parkin, can regulate mitophagy [14] . PINK1 is a cytosolic and mitochondrion-associated kinase that is continuously degraded in healthy cells by mitochondrial proteases, including the mitochondrial inner membrane protease Presenilin-associated, rhomboid-like (PARL) protein [15] , [16] . Mitochondrial membrane depolarization inhibits PINK1 degradation, causing it to accumulate and promote mitophagy via recruitment of another familial Parkinson's protein, the E3 ubiquitin ligase, parkin [17] , [18] . However, the detailed mechanism of PINK1 degradation and stabilization remains unclear. PINK1 is mutated in autosomal recessive early-onset Parkinson’s disease [19] , [20] , [21] , but many putative pathogenic mutations are found in heterozygous individuals or even in healthy controls [20] , which suggests that it is important to identify other critical factors for the protective effect of PINK1 against dopaminergic degeneration. Phosphoglycerate mutase family member 5 (PGAM5), paralog member 5 of a family of highly conserved phosphoglycerate mutases, is a 32 kDa mitochondrial protein that apparently lacks phosphotransfer function on phosphoglycerates, but retains activity as a serine/threonine protein phosphatase that regulates the ASK1 kinase [22] . The functions of PGAM5 are complex since it also serves as an antioxidant regulator in the Kelch ECH associating protein 1–nuclear factor-E2-related factor 2 signalling pathway and binds Bcl-X L [23] , [24] . Recently, PGAM5 was described as a downstream target of RIP3 responsible for recruiting the RIP1-RIP3-MLKL necrosis ‘attack’ complex to mitochondria [4] , [25] . Interestingly, PGAM5 has also been reported as a genetic suppressor of PINK1 in Drosophila [26] , as well as a substrate of PARL [27] . Thus, it is important to establish the in vivo role of PGAM5 in mitochondrial disease pathogenesis. Here we show PGAM5 is a new mitophagy regulator in the PINK1/parkin pathway, and that genetic deficiency of PGAM5 in mice causes a Parkinson’s disease-like phenotype. PGAM5 regulates PINK1/parkin mediated mitophagy We generated Pgam5 knockout (KO) mice from gene-targeted embryonic stem cells and verified that homozygotes exhibited a nearly complete loss of Pgam5 messenger RNA as well as protein expression ( Supplementary Fig. 1 ). Because of our interest in mitochondrial regulation, we examined mouse embryonic fibroblasts (MEFs) by transmission electron microscopy (TEM). We observed that KO MEFs contained an increased number of swollen bulbous mitochondria that lacked normal cristae and were filled with non-descript granular debris that were not found in wild-type (WT) MEFs ( Fig. 1a , and Supplementary Fig. 2a ). Moreover, KO MEFs manifested constitutively elevated levels of intracellular ROS and a subtle decrease in the mitochondrial potential measured by the dye TMRE, which indicates stressed or damaged mitochondria [4] ( Supplementary Fig. 2b,c ). We hypothesized that PGAM5 promotes the clearance of unhealthy or damaged mitochondria to maintain mitochondrial homeostasis through mitophagy. We therefore examined Pgam5 KO MEFs treated with carbonyl cyanide m -chlorophenyl hydrazone (CCCP), which exacerbates mitochondrial stress and mitophagy by uncoupling the mitochondrial proton gradient essential for oxidative phosphorylation [17] , [18] . After CCCP treatment, WT MEFs showed an increase in double-membrane vesicles, a decrease in mitochondria and some mitochondria encapsulated by a double-membrane structure (DMS) characteristic of mitophagy ( Fig. 1b ). By contrast, TEM of KO MEFs revealed increased numbers of swollen unhealthy mitochondria but double-membrane vesicles-encapsulated mitochondria were absent ( Fig. 1b and quantification in Supplementary Fig. 2d ). CCCP treatment also increased ROS levels and decreased mitochondria membrane depolarization to a greater extent in KO compared with WT cells consistent with failed mitophagy ( Supplementary Fig. 2e,f ). 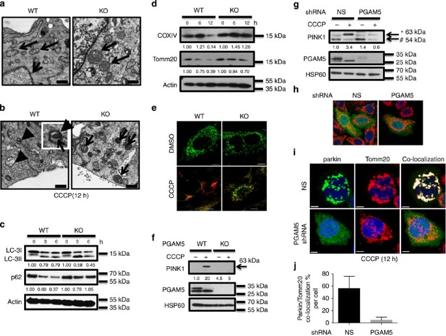Figure 1: PGAM5 is required for PINK1-triggered mitophagy. (a) WT andPgam5KO MEFs evaluated by TEM. The black arrows indicate mitochondria; (b) TEM analysis after 12 h CCCP treatment; black arrowheads indicate DMS. Inset shows a DMS with an encapsulated mitochondrion. The black arrows indicate mitochondria. Scale bar=0.5 micron; (c) WT and KO MEFs were treated with CCCP for 0, 3 or 6 h and cytosolic fractions were immunoblotted with anti-LC-3, anti-p62 or anti-actin as indicated. (d) Similar toc. Treated with CCCP for 6 and 12 h and immunoblotted for anti-COXIV, anti-Tomm20 or anti-actin as indicated. Forcandd, the numbers below each lane indicate the fractional band density compared with the 0 h time point, which has been set at 1.0; (e) Confocal photomicrographs of mt-Keima-transduced WT and KO MEFs treated with CCCP or DMSO vehicle for 12 h (six individual cells from each group were scanned and representative cells are shown); Intracellular mt-Keima excited at 450 nm was shown in green colour, while red colour indicated the excitation by 550 nm in the same cell. Scale bar=20 μm. (f) Mitochondrial extracts of WT andPgam5KO MEFs treated with DMSO (−) or CCCP (+) for 3 h and analysed by immunoblot as above. (Note that mouse PINK1 antibody can only detect the full-length PINK1). Arrow indicates the 63 kDa form of PINK1. (g) Hela cells transduced with either nonspecific (NS) or PGAM5 shRNA viruses were treated with CCCP for 3 h, and mitochondrial fractions were immunoblotted for the proteins indicated. Full-length (*63 kDa) and cleaved (#54 kDa) PINK1 are indicated. Forfandg, the numbers below indicate the full-length PINK1 band density compared with the first lane that has been set at 1.0 (h) Confocal micrographs of Hela cells as ingwere transfected with PARKIN-YFP (green) plasmid before CCCP treatment, then (i) treated with CCCP for 12 h. Mitochondria were stained with anti-Tomm20 (red) 4',6-diamidino-2-phenylindole stained nucleus was shown in blue. Co-localization was indicated by white colour. Scale bar=10 μm. (j) Quantification of the co-localization percentage of Tomm20 (red) with parkin (green) per cell by Imaris software (n=7 for NS andPGAM5shRNA group separately. Results are presented as mean and s.d. values and were analysed by the studentt-test). All the blots and images are representative of three independent experiments. DMSO, dimethylsulphoxide. Figure 1: PGAM5 is required for PINK1-triggered mitophagy. ( a ) WT and Pgam5 KO MEFs evaluated by TEM. The black arrows indicate mitochondria; ( b ) TEM analysis after 12 h CCCP treatment; black arrowheads indicate DMS. Inset shows a DMS with an encapsulated mitochondrion. The black arrows indicate mitochondria. Scale bar=0.5 micron; ( c ) WT and KO MEFs were treated with CCCP for 0, 3 or 6 h and cytosolic fractions were immunoblotted with anti-LC-3, anti-p62 or anti-actin as indicated. ( d ) Similar to c . Treated with CCCP for 6 and 12 h and immunoblotted for anti-COXIV, anti-Tomm20 or anti-actin as indicated. For c and d , the numbers below each lane indicate the fractional band density compared with the 0 h time point, which has been set at 1.0; ( e ) Confocal photomicrographs of mt-Keima-transduced WT and KO MEFs treated with CCCP or DMSO vehicle for 12 h (six individual cells from each group were scanned and representative cells are shown); Intracellular mt-Keima excited at 450 nm was shown in green colour, while red colour indicated the excitation by 550 nm in the same cell. Scale bar=20 μm. ( f ) Mitochondrial extracts of WT and Pgam5 KO MEFs treated with DMSO (−) or CCCP (+) for 3 h and analysed by immunoblot as above. (Note that mouse PINK1 antibody can only detect the full-length PINK1). Arrow indicates the 63 kDa form of PINK1. ( g ) Hela cells transduced with either nonspecific (NS) or PGAM5 shRNA viruses were treated with CCCP for 3 h, and mitochondrial fractions were immunoblotted for the proteins indicated. Full-length (*63 kDa) and cleaved (#54 kDa) PINK1 are indicated. For f and g , the numbers below indicate the full-length PINK1 band density compared with the first lane that has been set at 1.0 ( h ) Confocal micrographs of Hela cells as in g were transfected with PARKIN-YFP (green) plasmid before CCCP treatment, then ( i ) treated with CCCP for 12 h. Mitochondria were stained with anti-Tomm20 (red) 4',6-diamidino-2-phenylindole stained nucleus was shown in blue. Co-localization was indicated by white colour. Scale bar=10 μm. ( j ) Quantification of the co-localization percentage of Tomm20 (red) with parkin (green) per cell by Imaris software ( n =7 for NS and PGAM5 shRNA group separately. Results are presented as mean and s.d. values and were analysed by the student t -test). All the blots and images are representative of three independent experiments. DMSO, dimethylsulphoxide. Full size image We next performed biochemical analyses of mitophagy and found that although the microtubule-associated protein 1A/1B light chain 3 (LC-3) was processed from LC-3I to LC-3II, in both WT and KO MEF cells after 3 or 6 h of CCCP treatment, the autophagic removal of cytosolic sequestosome 1 (p62), was impaired in KO MEFs ( Fig. 1c ) [28] . With longer CCCP exposure (12 h), KO MEFs showed reduced mitochondrial clearance as indicated by the persistence of COX IV, an inner mitochondrial membrane (IMM) protein and Tomm20, an outer mitochondrial membrane (OMM) protein in total cell lysates ( Fig. 1d ). We directly visualized mitophagy using mt-Keima, an IMM-targeted fluorescent protein resistant to lysosomal proteases whose excitation fluorescence ( λ ex ) is 450 nm (green fluorescence) at neutral pH in the cytosol and shifts to 550 nm (red fluorescence) at acid pH following delivery of mitochondria to acidic lysosomes [29] . We observed that CCCP treatment of WT MEFs induced the expected shift of mt-Keima from an evenly distributed green mitochondrial appearance to a bright red punctate appearance, indicating relocation of mitochondria to acidic autolysosomes by mitophagy ( Fig. 1e , left panels). By contrast, Pgam5 KO cells exhibited persistent green fluorescence and very little red punctate fluorescence revealing a defect in mitophagy ( Fig. 1e , right panels, and quantification in Supplementary Fig. 2g ). Hence, PGAM5 is apparently indispensable for the process of mitophagy. Since PINK1 is a well-known mitophagy protein that binds PGAM5 (ref. 26 ), we tested its function in Pgam5 KO MEFs. We observed that purified mitochondria from WT cells treated with CCCP for 3 h exhibited stabilization of the 63 kDa full-length PINK1 protein but this effect was abolished in Pgam5 KO cells ( Fig. 1f ). Lentiviral-mediated expression of GFP-tagged PGAM5 in KO MEFs rescued PINK1 indicating that PGAM5 accounted for PINK1 mitochondrial stabilization ( Supplementary Fig. 3 ). We found that short hairpin RNA (shRNA) knockdown of PGAM5 in HeLa cells also disrupted PINK1 stabilization on the OMM after CCCP treatment ( Fig. 1g ). Notably, we also observed that CCCP shifted PGAM5 to a predominantly faster migrating species suggesting proteolytic cleavage in the mitochondria ( Fig. 1f,g ). Finally, parkin, which is recruited by PINK1 to assist mitophagy, was not influenced by the knockdown of PGAM5 under normal conditions ( Fig. 1h ). However, after CCCP treatment, parkin exhibited defective mitochondrial translocation and remained diffuse, likely due to impaired PINK1 stabilization and recruitment ( Fig. 1i,j for quantification). PGAM5 protects PINK1 from IMM degradation To investigate how PGAM5 regulates PINK1 stability, we first examined the phosphatase function of PGAM5 (ref. 22 ). We introduced a phosphatase-dead mutant (H105A) of PGAM5 into WT and KO MEFs and found that both the mutant and unaltered forms restored PINK1 stabilization following CCCP treatment indicating that PGAM5 phosphatase function was not essential ( Supplementary Fig. 4 ). We noticed that amino-terminal and carboxy-terminal-tagged PGAM5 protein showed two bands or one band, respectively, when exogenously expressed in HEK293T cells, confirming proteolytic cleavage occurs close to its N terminus ( Supplementary Fig. 5 ). In purified mitochondria from WT MEFs, we observed two endogenous PGAM5 bands, a 32 kDa band corresponding to full-length PGAM5, and another 3 kDa smaller consistent with previous observations that PGAM5 can be cleaved in the TM ( Fig. 2a left panel) [27] . Examining MEFs from mice genetically deficient in PARL, an IMM rhomboid protease, we observed that purified mitochondria only contained full-length PGAM5 confirming that it is a substrate of the IMM protease PARL and that PGAM5 is localized to the IMM ( Fig. 2a , right panel) [27] . We further confirmed the IMM location of PGAM5 by exposing purified mitochondria to increasing doses of proteinase K, which degrades outer membrane proteins such as Tomm20. PGAM5 resisted proteinase K degradation confirming an IMM location ( Fig. 2a ) [27] . Previously it has been shown that PINK1 undergoes cleavage by PARL and turnover in the IMM in healthy mitochondria [15] . Therefore, our data implied that PGAM5 facilitates stabilization of PINK1 against PARL cleavage in the IMM after CCCP exposure. This inference was strengthened by an experiment in which PARL expression was reduced by a small hairpin RNA (PARLsh) and we found that PINK1 was stabilized even in PGAM5 KO mitochondria following CCCP treatment ( Fig. 2b and Supplementary Fig. 6 ). 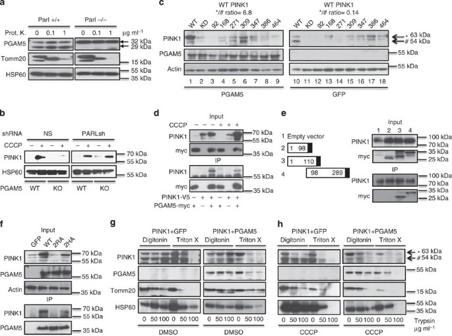Figure 2: PGAM5 stabilizes PINK1 in mitochondria. (a) Mitochondria from MEFs fromParlWT (+/+) and KO (−/−) mice were treated with the indicated doses of proteinase K (Prot.K) for 30 min on ice and then immunoblotted for the indicated proteins. Full-length and cleaved PGAM5 bands are indicated with arrows. (b)Pgam5WT and KO MEFs were transduced with either nonspecific (NS) orParlshRNA and either treated (+) or not (−) with CCCP for 3 h. Mitochondria were then purified and analysed by immunoblot for the indicated proteins. (c) WT PINK1 as well as kinase dead (KD) or Parkinson’s disease-associated PINK1 mutants (C92F, A168P, H271Q, G309D, L347P, G386S, R464H) were co-transfected into HEK293T cells with the same amount PGAM5 (lane 1–9) or GFP (lane 10–18) expression plasmids and total cell lysates were immunoblotting for PINK1, PGAM5 and actin. The ratio of WT full-length (63 kDa) versus cleaved (54 kDa) PINK1 (*/#) is shown. (d) Anti-myc immunoprecipitates (IP) of lysates from 293T cells transfected with combinations of myc-tagged PGAM5 and PINK1-V5 with or without CCCP treatment and immunoblotting with anti-PINK1 or anti-myc. (e) Four constructs expressing either: (1) no PGAM5 (empty vector) or (2) amino acids 1–98, (3) 1–110 and (4) 98–289 truncated versions of PGAM5 (left panel). Immunoblot of HEK293T cells expressing PINK1-GFP and myc-tagged PGAM5 truncation mutants as indicated with anti-PINK1 or anti-myc for the input proteins as well as the anti-GFP IP (right panel). (f) Co-transfection of GFP, WT PGAM5, 2RA mutant (R98A and R104A) or the 2HA mutant (H99A and H105A) with a PINK1 expression plasmid into HEK293T cells and the input cell lysates as well as the anti-myc IP were immunoblotted with antibodies against PINK1, PGAM5 or actin. WT PINK1 was expressed in HEK293T cells with or without PGAM5 or a GFP control plasmid after (g) DMSO or (h) CCCP treatment. Cells were permeabilized with digitonin or Triton X-100 separately, followed by treatment with the indicated amounts of trypsin on ice for 30 min. Cell lysates were immunoblotted for PINK1, PGAM5, Tomm20 or HSP60 as indicated. Full-length (*63 kDa) and cleaved (#54 kDa) PINK1 are shown. Figure 2: PGAM5 stabilizes PINK1 in mitochondria. ( a ) Mitochondria from MEFs from Parl WT (+/+) and KO (−/−) mice were treated with the indicated doses of proteinase K (Prot.K) for 30 min on ice and then immunoblotted for the indicated proteins. Full-length and cleaved PGAM5 bands are indicated with arrows. ( b ) Pgam5 WT and KO MEFs were transduced with either nonspecific (NS) or Parl shRNA and either treated (+) or not (−) with CCCP for 3 h. Mitochondria were then purified and analysed by immunoblot for the indicated proteins. ( c ) WT PINK1 as well as kinase dead (KD) or Parkinson’s disease-associated PINK1 mutants (C92F, A168P, H271Q, G309D, L347P, G386S, R464H) were co-transfected into HEK293T cells with the same amount PGAM5 (lane 1–9) or GFP (lane 10–18) expression plasmids and total cell lysates were immunoblotting for PINK1, PGAM5 and actin. The ratio of WT full-length (63 kDa) versus cleaved (54 kDa) PINK1 (*/#) is shown. ( d ) Anti-myc immunoprecipitates (IP) of lysates from 293T cells transfected with combinations of myc-tagged PGAM5 and PINK1-V5 with or without CCCP treatment and immunoblotting with anti-PINK1 or anti-myc. ( e ) Four constructs expressing either: (1) no PGAM5 (empty vector) or (2) amino acids 1–98, (3) 1–110 and (4) 98–289 truncated versions of PGAM5 (left panel). Immunoblot of HEK293T cells expressing PINK1-GFP and myc-tagged PGAM5 truncation mutants as indicated with anti-PINK1 or anti-myc for the input proteins as well as the anti-GFP IP (right panel). ( f ) Co-transfection of GFP, WT PGAM5, 2RA mutant (R98A and R104A) or the 2HA mutant (H99A and H105A) with a PINK1 expression plasmid into HEK293T cells and the input cell lysates as well as the anti-myc IP were immunoblotted with antibodies against PINK1, PGAM5 or actin. WT PINK1 was expressed in HEK293T cells with or without PGAM5 or a GFP control plasmid after ( g ) DMSO or ( h ) CCCP treatment. Cells were permeabilized with digitonin or Triton X-100 separately, followed by treatment with the indicated amounts of trypsin on ice for 30 min. Cell lysates were immunoblotted for PINK1, PGAM5, Tomm20 or HSP60 as indicated. Full-length (*63 kDa) and cleaved (#54 kDa) PINK1 are shown. Full size image We therefore examined the ability of PGAM5 to stabilize WT PINK1 as well as a variety of PINK1-mutant alleles causing recessive early-onset Parkinson’s disease. We co-expressed epitope-tagged versions of PGAM5 and PINK1, and we found that the presence of PGAM5 increased the level of full-length WT PINK1 (*63 kDa) and decreased the PARL-cleaved form of PINK1 (#54 kDa) ( Fig. 2c ). By contrast, co-expression with a GFP control protein left WT PINK1 as a weak full-length band together with smaller PARL-cleaved bands ( Fig. 2c , compare lanes 1 with 10 in which the ratios of the 63 to 54 kDa PINK1 forms were 6.8 and 0.14, respectively) [15] . However, the Parkinson-associated mutant forms of PINK1 exhibited poor stability and varied cleavage patterns ( Fig. 2c , lanes 11–18). Moreover, PGAM5 overexpression failed to increase the accumulation of full-length versions of the mutant proteins with the possible exception of 309 ( Fig. 2c , lanes 2–9). The stabilization of PINK1 by PGAM5 in this co-expression assay is not affected by CCCP treatment ( Supplementary Fig. 7 ). Therefore, Parkinson-associated PINK1 mutants are generally resistant to PGAM5 stabilization. We tested the mechanism of stabilization by examining the importance of direct association of PGAM5 with PINK1. We found that myc-tagged PGAM5 co-precipitated PINK1 in HEK293T cells and this was moderately diminished by CCCP treatment ( Fig. 2d ). Co-immunoprecipitation of fragments of PGAM5 with GFP-tagged PINK1 demonstrated that the 1–110 fragments or the 98–289 fragments bound PINK1, but the 1–98 fragments did not, implying that residues 98–110 of PGAM5 were important for binding ( Fig. 2e ). Alignment of PGAM5 amino-acid sequences from different species showed that this region (98–110) is highly evolutionarily conserved with an amino-acid motif consisting of two RH dipeptides precisely separated by four hydrophobic amino acids (the ‘di-RH’ motif) (see Supplementary Fig. 8 for a protein sequence alignment). We therefore created amino-acid substitutions of either both arginines (2R) or both histidines (2H) with alanine and expressed these two PGAM5 mutants 2RA (R98A/R104A) and 2HA (H99A/H105A) at equivalent levels to the WT protein and tested for PINK1 stabilization. We found the 2RA mutation lost essentially the entire PINK1 stabilization function ( Fig. 2f ) and the corresponding immunoprecipitation experiment showed that PGAM5 2RA completely lost the ability to bind to PINK1 ( Fig. 2f ). Furthermore, we found that the 2H mutant showed a partial loss of PINK1 stabilization and a corresponding partial loss of association with PINK1 ( Fig. 2f ). This supports the view that direct association between PGAM5 and PINK1 is crucial for the stabilization of the latter protein and also demonstrates that the di-RH motif is important for this association. Notably, PINK1 stabilized on purified mitochondria by CCCP treatment, becomes sensitive to exogenously added proteases implying that it traffics to the OMM whereas PGAM5 is protected implying that remains in the IMM ( Supplementary Fig. 9 ). This could account for the partially diminished binding of PINK1 to PGAM5 after CCCP treatment ( Fig. 2d ). We therefore assessed PINK1 topology by transfecting PINK1 with or without PGAM5 into HEK293T cells and then gently permeabilizing the plasma membrane with digitonin, which does not compromise the OMM or IMM [30] . We then added trypsin, which diffuses into the cytosol and cleaves OMM proteins and found that with no CCCP treatment, PINK1 (both full-length and cleaved forms) and PGAM5 were protected from degradation and therefore located in the IMM ( Fig. 2g ). Furthermore, PGAM5 but not GFP co-expression could stabilize the full-length 63 kDa version of PINK1. Control treatment with Triton X-100, which will permeabilize the mitochondrial as well as plasma membranes, permitted both PINK1 and PGAM5 to be degraded by trypsin. After CCCP treatment, we observed that full-length 63 kDa PINK1 was enhanced by PGAM5 but not GFP co-expression and specifically re-located to the OMM as reflected by trypsin sensitivity after digitonin ( Fig. 2h ). The 54 kDa and smaller bands of PINK1 observed in the GFP control samples, remained resistant to trypsin in the digitonin samples ( Fig. 2h , left panels). All species of PINK1 became sensitive to trypsin after Triton X-100 treatment. These data confirm PINK1 is localized first in the IMM, and that PGAM5 serves as a selective gateway to the OMM for the full-length 63 kDa form of PINK1 but not the lower molecular weight cleaved forms. In response to mitochondrial dysfunction induced by CCCP treatment, it appears that full-length PINK1 selectively and transiently associates with PGAM5, which enables transfer to the OMM where it takes up residence to initiate mitophagy. PGAM5 itself remains in the IMM. We summarized this as an ‘inside-out’ translocation pathway of PINK1 ( Fig. 3 ). Thus, mitochondria membrane depolarization alone is not sufficient to stabilize PINK1 on the mitochondria to initiate mitophagy, but PGAM5 is also specifically required for the selective stabilization of full-length PINK1. 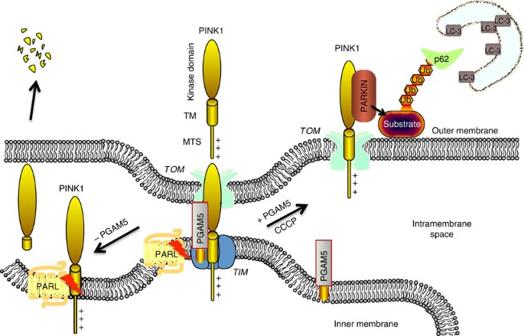Figure 3: Inside-out PINK1 translocation model. PGAM5 is an IMM protein that protects PINK1 from degradation by mitochondrial proteases including PARL. After CCCP treatment, full-length PINK1 protected by PGAM5 will move to the OMM, while PGAM5 remains on the IMM. In the absence of PGAM5, PINK1 loses the protection from PGAM5, and will be cleaved and degraded. CCCP can trigger PGAM5 stabilized PINK1 translocation from IMM to OMM where it associates with parkin leading to ubiquitination events associated with p62 recruitment and culminating in LC-3-mediated mitophagy. Figure 3: Inside-out PINK1 translocation model. PGAM5 is an IMM protein that protects PINK1 from degradation by mitochondrial proteases including PARL. After CCCP treatment, full-length PINK1 protected by PGAM5 will move to the OMM, while PGAM5 remains on the IMM. In the absence of PGAM5, PINK1 loses the protection from PGAM5, and will be cleaved and degraded. CCCP can trigger PGAM5 stabilized PINK1 translocation from IMM to OMM where it associates with parkin leading to ubiquitination events associated with p62 recruitment and culminating in LC-3-mediated mitophagy. Full size image Aged PGAM5 KO mice show a Parkinson’s-like movement disorder PINK1-deficient mice show some features reminiscent of Parkinson’s disease, with decreased DA levels in the brain and reduced motor activity, but dopaminergic neurons do not degenerate in large numbers [31] , [32] . Recently, it has been proposed that one cellular role of PINK1 is to mediate mitophagy [8] , [14] , and this and other mitochondrial processes may become defective with age in Parkinson’s disease [5] , [8] , [9] , [13] , [14] . Hence, we evaluated neurological function using behavioural tests on Pgam5 KO mice (female, WT n =10, KO n =8) at 1 year of age [33] , [34] . The body weight and general health were comparable between WT and KO mice ( Fig. 4a ). In the open-field test, we observed that KO mice show a significant reduction in the overall locomotor activity compared with WT littermates, including reduced time spent mobile and shorter total distance travelled ( Fig. 4b , left and middle panel), especially in the centre of the testing arena ( Fig. 4b , right panel). Gait analysis data revealed that KO mice had shorter hind limb stride length, increased stride frequency and increased step angle variability ( Fig. 4c ), which resembles a Parkinsonian gait [33] , [34] . Furthermore, the Pgam5 KO mice showed a reduction in total number of rears during a cylinder observational test ( Fig. 4d ); an increased time to move all four limbs in the akinesia test ( Fig. 4e ); and increased traversal time to cross a horizontal ladder ( Fig. 4f ). In the vertical pole test for the assessment of balance and coordination, the KO mice took longer to turn their bodies 180 degrees from the head up start position before descending the pole ( Fig. 4g , left panel), but there was no significant difference between KO and WT mice in time to descend the pole ( Fig. 4g , right panel). In summary, KO mice show impaired movement function, manifested as Parkinsonian gait changes, bradykinesia and an overall reduction in movement initiation, while lacking an overt defect in balance and coordination on the pole test as well as rotarod test ( Supplementary Fig. 10 ). In conclusion, at 1 year of age, the behavioural phenotype of Pgam5 KO mice reveals some, but not all Parkinson’s disease features. 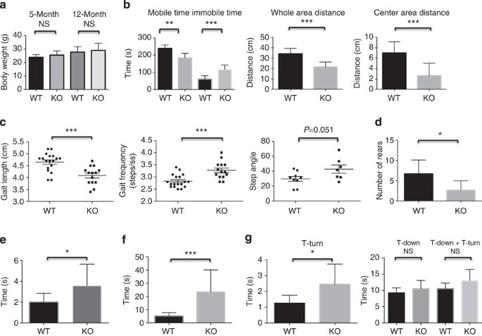Figure 4: AgedPgam5KO mice show a Parkinson’s disease-like phenotype. (a) Body weight was measured in 5-month-old and 12-month-old femalePgam5WT and KO mice. Behavioral measurements on 12-month-old female WT and KO mice (WTn=10, KOn=8) were as follows: (b) Open-field tests including time spent mobile, time spent immobile, whole area distance and centre area distance; (c) Gait length, gait frequency in steps/ss and step angle; (d) rearing test, (e) akinesia test and (f) ladder climb test and (g) vertical pole test. T-turn indicates the time mice spent to turn their bodies 180 degrees from the head up start position before descending the pole. T-down indicates the time mice spent to descend to the bottom of pole. Graphs show the mean and s.d. values and were analysed by the student’st-test, *P<0.05, **P<0.01, ***P<0.001, NS, not significant. Figure 4: Aged Pgam5 KO mice show a Parkinson’s disease-like phenotype. ( a ) Body weight was measured in 5-month-old and 12-month-old female Pgam5 WT and KO mice. Behavioral measurements on 12-month-old female WT and KO mice (WT n =10, KO n =8) were as follows: ( b ) Open-field tests including time spent mobile, time spent immobile, whole area distance and centre area distance; ( c ) Gait length, gait frequency in steps/ss and step angle; ( d ) rearing test, ( e ) akinesia test and ( f ) ladder climb test and ( g ) vertical pole test. T-turn indicates the time mice spent to turn their bodies 180 degrees from the head up start position before descending the pole. T-down indicates the time mice spent to descend to the bottom of pole. Graphs show the mean and s.d. values and were analysed by the student’s t -test, * P <0.05, ** P <0.01, *** P <0.001, NS, not significant. Full size image PGAM5 deficiency causes mouse DA neuron degeneration To determine whether the abnormal movement phenotype in Pgam5 KO mice might be due to dopaminergic dysfunction, we examined DA, and its metabolites dihydroxyphenylacetic acid, 3-methoxytyramine and homovanillic acid neurochemistry in striatal lysates by high-performance liquid chromatography (HPLC) with electrochemical detection (in mice at 1 month, 2 months and 12 months of age). We observed that the KO and WT mice showed no difference in neurotransmitter levels at 1 month of age. Starting from 2 months old, we found a mild but significant decrease of DA content in KO compared with WT mice ( Fig. 5a ). The DA and its metabolic product of dihydroxyphenylacetic acid were also significantly reduced in 12-month-old KO mice ( Fig. 5b ). However, the levels of other metabolites of 3-methoxytyramine and homovanillic acid were equivalent in KO and WT animals at all time points ( Fig. 5c,d ). To analyse whether the catabolism of DA is altered in WT versus KO mice, we calculated the DA turnover ratio and we observed no significant changes in any time point ( Supplementary Fig 11a,b ). Further analyses also did not show any significant changes in serotonin (5HT), 5-hydroxyindoleacetic acid and 5HT turnover ratio ( Supplementary Fig. 11c–e ). 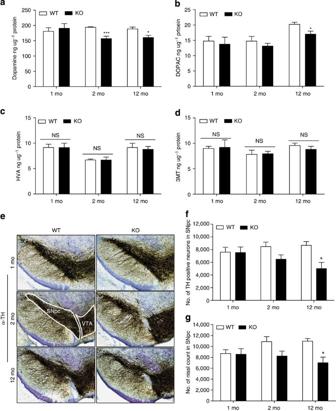Figure 5:Pgam5KO mice show progressive dopaminergic neurodegeneration. High-performance liquid chromatography-electrochemical detection quantitation of (a) striatal DA and its metabolites (b) dihydroxyphenylacetic acid (DOPAC) (c) Homovanillic acid (HVA) and (d) 3MT levels at three different time points (1, 2 and 12-month-old) inPgam5WT or KO mice. In 1, 2 and 12 mo cohorts, TH-positive neurons were quantified in the SNpc region of WT and KO mice by unbiased stereological counting. (e) Representative images of TH-immunohistochemistry from WT and KO mice. The VTA region is indicated. Stereological quantitation of (f) TH and (g) Nissl-positive neurons in the SNpc (n=4 mice per group). Error bars represent the mean±s.e.m.,n=4 mice per group. (two-way analysis of variance, ***P<0.01, *P<0.05, NS, not significant). mo, month old. Figure 5: Pgam5 KO mice show progressive dopaminergic neurodegeneration. High-performance liquid chromatography-electrochemical detection quantitation of ( a ) striatal DA and its metabolites ( b ) dihydroxyphenylacetic acid (DOPAC) ( c ) Homovanillic acid (HVA) and ( d ) 3MT levels at three different time points (1, 2 and 12-month-old) in Pgam5 WT or KO mice. In 1, 2 and 12 mo cohorts, TH-positive neurons were quantified in the SNpc region of WT and KO mice by unbiased stereological counting. ( e ) Representative images of TH-immunohistochemistry from WT and KO mice. The VTA region is indicated. Stereological quantitation of ( f ) TH and ( g ) Nissl-positive neurons in the SNpc ( n =4 mice per group). Error bars represent the mean±s.e.m., n =4 mice per group. (two-way analysis of variance, *** P <0.01, * P <0.05, NS, not significant). mo, month old. Full size image To investigate the effect of PGAM5 deficiency on DA neuron viability, we quantified tyrosine hydroxylase (TH) immunoreactivity and Nissl staining in the substantia nigra pars compacta (SNpc) and ventral tegmental area (VTA) by an unbiased stereological method. WT and KO mice exhibited no difference in TH-positive or Nissl-stained neurons number at 1 month old, which indicates that early development is normal in the absence of PGAM5. At 2 months of age, there is a trend towards the loss of TH-positive and Nissl-stained neurons. At 12 months of age, we observed a significant loss of TH-positive (43%) and Nissl (35%) stained neurons in the SNpc ( Fig. 5e–g ). Stereological counts from the VTA did not show any significant changes in TH- and Niss-positive neurons at any age ( Supplementary Fig. 11f,g ). Thus, VTA DA neurons are less sensitive than SNpc DA neurons to the absence of PGAM5, which is similar to the differential vulnerability of these DA neurons in Parkinson’s disease. L-3,4-dihydroxyphenylalanine (L-DOPA) is the precursor of DA and an effective treatment to rescue the behavioural abnormalities in Parkinson’ disease. We administered L-DOPA to 18-month-old WT and KO mice, and observed increased mobility and activity in KO mice in the open-field test. We found a mild increase in the movement of the WT mice (probably due to the high dose of L-DOPA injected into aged mice), but a much more notable improvement in the mobility and activity of the KO mice after treatment with L-DOPA ( Fig. 6a,b ). We also evaluated other regions of the brain from Pgam5 KO mice. No obvious general neurodegeneration was observed in the cortex, hippocampus or cerebellum ( Supplementary Fig. 12 ). Collectively, these data indicate that the abnormal behaviour phenotype of the KO mice likely involves the documented loss of SNpc DA neurons. Finally, we evaluated heart tissue from Pgam5 KO mice, since PINK1 was has been reported to be important for heart function [35] . We did not observe a mitochondrial abnormality in heart tissue by TEM in PGAM5 KO mice ( Supplementary Fig. 13 ). Thus, mice genetically deficient in PGAM5 exhibit a specific neurological abnormality related with progressive loss of SNpc DA neurons, which mimics a Parkinsonian-like behavioural phenotype. 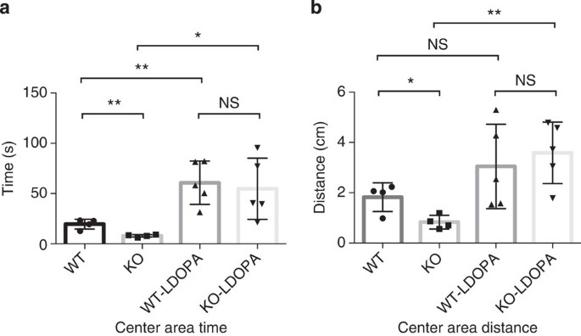Figure 6: L-DOPA rescues the abnormal behaviour phenotype in KO mice. The 18-month-oldPgam5WT and KO mice received either water as control (n=4), or 5 mg kg−1L-DOPA and 12.5 mg kg−1Benserazide (n=5) by intraperitoneal injection. Twenty minutes later, mice were subjected to the open-field test and the centre area time in seconds (s) as well as the centre area distance in centimeters (cm) were measured as described in the Materials and Methods. Graphs show the mean and s.d. values and were analysed by the studentt-test, NS, no significance; *P<0.05; **P<0.01. Figure 6: L-DOPA rescues the abnormal behaviour phenotype in KO mice. The 18-month-old Pgam5 WT and KO mice received either water as control ( n =4), or 5 mg kg −1 L-DOPA and 12.5 mg kg −1 Benserazide ( n =5) by intraperitoneal injection. Twenty minutes later, mice were subjected to the open-field test and the centre area time in seconds (s) as well as the centre area distance in centimeters (cm) were measured as described in the Materials and Methods. Graphs show the mean and s.d. values and were analysed by the student t -test, NS, no significance; * P <0.05; ** P <0.01. Full size image Our studies have shed light on the mechanism of PINK1 stabilization by unveiling a function of the mitochondrial regulatory protein PGAM5. PINK1 stabilization and subsequent parkin recruitment triggers mitophagy, which selectively eliminates dysfunctional mitochondria to protect cells/tissues from oxidative stress and cell death [13] , [14] . Here we provide evidence suggesting that mitophagy may contribute to dopaminergic neurodegeneration and movement disorders in experimental animals by the role of PGAM5 in these processes. PINK1 and parkin also regulate mitochondrial quality control through other pathways including mitochondria fusion/fission and biogenesis, to which PGAM5 may also contribute [36] , [37] . Contrary to a previous study in Drosophila [26] , we found PGAM5 protects DA neurons from degeneration, presumably by promoting PINK1 stabilization. Consistent with a mitochondrial pathogenesis for Parkinson’s disease, PINK1 deficiency in Drosophila causes energy depletion, shortened lifespan and DA neuron degeneration [38] , [39] . Aged Pink1 -deficient mice show impaired neural activity similar to Pgam5 KO mice, but without DA neurodegeneration [32] ; and mutations in PINK1 and parkin predispose to the movement disorders and DA neurodegeneration that characterizes familial Parkinson’s disease in humans [20] . The role for the mitochondrial protein PGAM5 in DA neuron pathology, lends further weight to the mitochondrial theory of Parkinson’s pathogenesis. The Pgam5 KO mice showed a movement disorder at 1 year of age, as well as dopaminergic neurodegeneration at an even earlier age. However, the magnitude of DA loss in Pgam5 KO mice is very small. In humans and in MPTP-treated mice, a loss of at least 75–80% of the DA neurons is required for locomotor problems to be exhibited [40] . The relatively small decrease of DA may be due to the compensatory secretion of DA from remaining DA neurons in SN or VTA. Another possibility is that the movement disorder phenotype may also result from dysfunctional DA neurons, a decrease of DA receptor sensitivity or other neurotransmitter systems, which have not yet been identified in Pgam5 KO mice. An important question is why Pgam5 KO mice apparently show a more severe phenotype than the PINK1 KO mouse [31] , [32] . We hypothesize that the difference between Pink1 KO and Pgam5 KO may be due to microbiome differences, uncontrolled environmental variables or genetic background differences. Recent discoveries clearly showed that mouse microbiota modulate neuron development [41] . Mice from different facilities and vendors also bear quite different intestinal microbiota [42] , which may influence the assessment of neurological function. Mouse genetic background also impacts the results of mouse KO models, since the accumulation of homozygous mutations during the inbreeding may disrupt proteins whose function is important for the evaluated mouse phenotype. For example, a point mutation in C56Bl6/N inbred mice strain attenuates the sensitivity to cocaine responses [43] . Moreover, the autonomous deletion of Casp11 in stain 129 mice reduces inflammasome activation compared with C57Bl6 strain [44] . Alternatively, the different outcomes may be due to the lack of compensatory mechanisms in the Pgam5 KO mice, which are active in Pink1 KO mice. We remain open to the possibility that PGAM5 may regulate other factors essential for DA neuron survival independent of the PINK1/parkin pathway. We have not observed any direct effect of PGAM5 on the mitochondrial import mechanism; however, there may be indirect effects on import as well as on the mitochondria fission/fusion system regulated by Drp1 (ref. 25 ). Previous reports have mentioned, and we also confirmed (data not shown), that PGAM5 strongly interacts with KEAP1, which is an adaptor protein for E3 ubiquitin ligase CUL3. PGAM5 can help release NRF2 from KEAP1, to facilitate NRF2-regulated antioxidant gene expression. Lack of PGAM5 disrupts both PINK1/parkin-mediated mitophagy and the NRF2-regulated antioxidant response, which could account for the DA neuron degeneration [23] . These additional factors might explain why DA neurodegeneration is absent in Pink1/Parkin KO mice but present in the Pgam5 KO mice. Homozygous recessive and compound heterozygote mutations in PINK1 have been identified in 1–2% of early-onset Parkinson’s disease patients [45] . PGAM5 mutations have not yet been reported in any human disease and whether PGAM5 mutations can be found in unexplained familial Parkinson’s disease patients now becomes a question of great interest. Patients with germline mutations in PINK1 or parkin show a restricted degeneration of DA neurons with no general neurodegeneration or abnormalities in other tissues. Pgam5 KO mice show an analogous restricted phenotype. It is unclear why only DA neurons, rather than other types of cells, are sensitive to the PINK1/parkin mutations or PGAM5 deficiency. The fact that DA neurons require energy generated from mitochondria and that DA neurons in SNc are quite sensitive to the oxidative stress generated from mitochondria might explain why maintaining healthy mitochondria is crucial for DA neuron viability [46] . PGAM5 deficiency fails to scavenge oxidative stress and abnormal mitochondria, which apparently leads to specific dopaminergic neuron degeneration. In conclusion, our data indicate that PGAM5 is a regulator of mitophagy involved in mitochondrial turnover and a key determinant of DA neuron survival in vivo . The Pgam5 KO mouse may be useful for the development of diagnostic tests and drug discovery for Parkinson’s disease in the future. Mice and cells Validated Pgam5 gene-targeted ES cells (B6 background: JM8.N4) were purchased from the European Mouse Mutant Cell Repository and chimeric mice were derived by microinjection of ES cells into blastocyst donors. Pgam5 KO mice were generated by breeding chimeric animals (Laboratory Animal Service Program of NCI-Frederick). Pgam5 WT and KO mice were bred and maintained in NIH animal facility at SPF (specific pathogen-free) conditions. Mouse experiments were carried out in accordance with NIAID Animal Care and Use Committee guidelines under an approved protocol. Twelve-month old female mice were used in all the animal study unless specifically indicated. MEF cells were prepared from day 12.5 embryos and cultured in DMEM/F12 full media (FM) (FM: 10% fetal bovine serum, 4 mM L -glutamine, 100 IU ml −1 penicillin and 100 mg ml −1 streptomycin) plus nonessential amino acids. Bone marrow cells were cultured in RPMI FM plus 20 ng ml −1 mouse M-CSF (Biolegend) for 7 days to induce macrophage differentiation. Parl WT and KO MEFs are from Dr Bart De Strooper (Centre for Human Genetics, Flanders Interuniversity Institute for Biotechnology (VIB4) and K.U. Leuven, Leuven, Belgium). Reagents The homemade PGAM5 antibody was made against the peptide, CGSLEKDRTLTPLGR by Genscript (NJ, USA). Commercial PGAM5 antibody was purchased from Abcam (Ab126534). Mouse PINK1 and PARL (Sigma); Human PINK1 (Novus) and LC-3, COXIV, VDAC, Actin, HSP60 and myc-tag antibodies (Cell Signaling Technology). Primary antibodies were used at 1:1,000 dilution in 5% non-fat milk, while HRP-labelled secondary antibodies (Southern Biotech) were used at 1:4,000 dilution. PGAM5 siRNA sequence: 5′- ACGCGCGCCAUAGAGACCACCGAUA -3′ (Life Technology, stealth siRNA). Pgam5 real-time PCR primers, forward: 5′- ATCTGGAGAAGACGAGTTGACA -3′; reverse: 5′- CCTGTTCCCGACCTAATGGT -3′. Lentiviral shRNA-mediated knockdown and cDNA overexpression pLKO.1 PGAM5 shRNA plasmids were purchased from Open Biosystem/Thermo Scientific. MEF cells were infected with lentivirus encoding shRNA against PGAM5 for 24 h before selection with 10 μg ml −1 puromycin according to the manufacturer’s specifications. The PGAM5 sequence was cloned into bicistronic lentiviral GFP vectors (abmgood). GFP control virus and PGAM5-GFP lentivirus were used to transduce MEF cells followed by puromycin selection as above. Western blot Cells were collected and lysed in buffer (20 mM Tris/HCl, pH 7.2, 0.5% (v/l) Nonidet P-40, 300 mM NaCl, 3 mM EDTA, 3 mM EGTA, 2 mM dithiothreitol, 2 mM PMSF, 100 μM leupeptin, 10 μM bestatin, 10 μM pepstatin and 2 μg ml −1 of aprotinin). Supernatants were collected after centrifugation at 10,000 g for 20 min at 4 °C, separated by 4–20% SDS–polyacrylamide gel electrophoresis and analysed by immunoblot. Cells and tissue mitochondria were purified by using Qproteome mitochondria isolation Kit (Qiagen). The mitochondria pellet was then lysed in 2 × SDS loading buffer and loaded onto SDS–polyacrylamide gel electrophoresis gels for western blot. The quantification of western blot bands as well as representative examples of uncropped western blots are included in Supplementary Fig. 14 ). Live cell imaging MEFs stably transduced with lentivirus encoding mitochondria-targeted Keima protein (mt-Keima) were cultured in glass-bottom dishes (MatTek). Cells were always kept around 50% confluency before any treatment. Cells were treated with 20 μM CCCP for 24 h and then scanned and images were collected on a Leica TCS-NT/SP confocal microscope (Leica Microsystems, Exton, PA USA) using a × 40 oil immersion objective NA 1.32. Detector slits were configured to minimize any cross-talk between the channels. Images were processed using the Leica TCS-NT/SP software (version 1.6.587), Imaris 3.2 (Bitplane AG, Zurich, Switzerland), and analysed and quantified by ImageJ software. Trypsin protection assay Transfected cells or purified mitochondria were resuspended in cold Hank’s balanced salt solution or mitochondria storage buffer (Qiagen mitochondria isolation kit). Cells were first treated with 20 μM digitonin or 0.05% Triton X-100 for 1 min, and then cells (or purified mitochondria) were incubated with different concentrations of trypsin on ice for 30 min. A quantity of 6X SDS loading dye was added to stop the reaction and lyse the cells (mitochondria) for western blot analysis. Behaviour tests The movement of Pgam5 KO and WT mice (WT n =10, KO n =8, all female, 12-month-old) was assessed in an open-field chamber. Mice were individually placed in a 50 × 50 cm square arena with 50 cm high black opaque plastic walls. The movement and activity of the mice were recorded for 60 min using a ceiling mounted video camera and a video mouse behavioural tracking system (Anymaze, Stoelting, Illinois). The open-field tests were performed during the dark phase of the light cycle. For gait assessment, video recordings of the underside of mice ambulating at a constant speed (13 and 18 cm s −1 ) were obtained using a transparent treadmill belt positioned above a high-speed digital camera (DigiGait Imaging System, Mouse Specifics, Boston MA). Video captures of 3–4 continuous seconds in which the mice walked without stumbling and maintained a consistent position on the belt for a minimum of 10 consecutive strides were subsequently analysed for multiple spatial and temporal gait parameters through the DigiGait Image Analysis System software. The DigiGait Imaging and Analysis system is based on ventral plane videography, and proprietary software that digitizes paw images and calculates the areas of approaching and retreating paws relative to belt and camera frame by frame as previously described [47] , [48] . Motor coordination was evaluated using a Rotamex-5 four-lane Rotarod (Columbus Instruments, Columbus OH) consisting of a 3 cm diameter ridged plastic rotary rod positioned 60 cm above the table. On day 1, the mice were acclimated to the testing environment by placing them on the stationary rotary rod. The mice received three 60-s acclimation trails separated by a 1 h rest interval. Mice were trained on a rotating rod starting the same afternoon by habituation to a slowly rotating rod (5 r.p.m.) for three 120-s trials with a 1 hour rest interval and on day 2, they received three 120-s training trials at the fixed speeds of 8 r.p.m. in the morning and 10 r.p.m. in the afternoon. The testing phase occurred 24 h after training. The mice were tested for 2 days at fixed rotation speeds, receiving three 120-s trials with 1 hour rests intervals between trials. On day 1, they were tested at 8 r.p.m., followed by 10 r.p.m. in the afternoon, and on day 2, they were tested at 12 r.p.m. in the morning and 15 r.p.m. in the afternoon. On day 3, the mice were placed on a rod programmed to accelerate from 4–40 r.p.m. The testing session consisted of three 300-s trials separated by 1 h rest intervals. Testing was spaced out over multiple days to prevent fatigue, or handling stress to confound the testing results. Latency to fall off the rotating rod was detected by photodetectors and automatically recorded along with the acceleration speed at the time of falling. Balance and coordination was also investigated using the vertical pole test as described by Matsuura et al . [49] Briefly, the mice were placed head up on a 50 cm high, 10 cm diameter vertical pole. The time for the mice to turn to a head downward position and the time to descend the pole were recorded and averaged over three trials. A number of neuromuscular phenotyping screens were also performed including the observation of rearing behaviour of mice placed in a transparent glass walled enclosure during a 90-s observational trial, the adhesive dot removal test in which the average time to remove a sticker placed on the snout was recorded over three trials, the akinesia test for the detection of mobility deficits as assessed by the latency to move all four limbs after placement onto a flat surface and a catalepsy test to assess the ability of the mice to correct an abnormally imposed body position after placement of the hind limbs on a raised 1.5-inch block by the experimenter. Finally, the mice were timed as they performed a ladder traversal test. The average time to cross a 30 cm long metal grid, with horizontally oriented bars placed 1.25 cm apart and positioned vertically at a 50° angle was calculated over three trials. All animal experiments were performed in accordance and with approval from the NHLBI and NIAID Animal Care and Use Committee. Monoamine analysis Biogenic amine concentrations were measured by HPLC with electrochemical detection [50] . Briefly, mice were killed by decapitation and the striatum was quickly removed. Striatal tissue was weighed and sonicated in 0.2 ml ice cold 0.01 mM perchloric acid containing 0.01% EDTA and 60 ng 3,4-dihydroxybenzylamine as an internal standard. After centrifugation (15,000 g , 30 min, 4 °C), the supernatant was passed through a 0.2 μm filter. Twenty microliters of the supernatant were analysed in the HPLC column (3 mm × 150 mm C-18 reverse phase column, Acclaim Polar Advantage II, Thermo Scientific, USA) by a dual channel coulochem III electrochemical detector (Model 5300, ESA, Chelmsford, MA, USA). The protein concentrations of tissue homogenates were measured using the BCA protein assay kit (Pierce, Rockford, IL, USA). Data were normalized to protein concentrations and expressed in ng ug −1 protein. Immunohistochemistry and quantitative analysis Mice were perfused with ice-cold phosphate-buffered saline (PBS) followed by 4% paraformaldehyde/PBS (pH 7.4). Brains were removed and post-fixed for 4 h in the same fixative. After cryoprotection in 30% sucrose/PBS (pH 7.4), the brains were frozen and serial coronal sections (60 μm sections) were cut with a microtome. Free-floating 60 μm sections were blocked with 5% goat serum/PBS plus 0.2% Triton X-100 and incubated with an antibody against TH (rabbit polyclonal; Novus Biologicals) followed by incubation with biotin-conjugated anti-rabbit antibody (anti-rabbit polyclonal; Vector Labs), ABC reagents (Vector Labs), and SigmaFast DAB Peroxidase Substrate (Sigma-Aldrich). Sections were counterstained with Nissl (0.09% thionin). As described before [50] , TH-positive cells and Nissl from the SNpc and VTA region were counted through optical fractionators, the unbiased, 3-diamensional method for cell counting. This method was carried out by using a computer-assisted image analysis system consisting of an Axiophot photomicroscope (Carl Zeiss Vision) equipped with a computer controlled motorized stage (Ludl Electronics), a Hitachi HV C20 camera and Stereo Investigator software (MicroBright-Field). The total number of TH-stained neurons and Nissl counts were calculated. Benserazide and L-DOPA treatment Nine 18-month-old WT and Pgam5 KO mice were divided into two groups receiving either intraperitoneal injections of 12.5 mg kg −1 benserazide (Sigma) 20 min before receiving intraperitoneal injections of 5 mg kg −1 L-DOPA (Sigma) or two injections of water separated by 20 min. Behavioural testing began 20 min after the L-DOPA injection [51] . Statistical analysis All histology quantitative data are expressed as the mean±s.e.m. Statistical significance was determined by two-way analysis of variance followed by Bonferroni post hoc analysis for comparison among multiple treatment groups. P values lower than 0.05 were considered to be significant. Respective P values are indicated in figure legends. Asterisks sign (*) indicate statistical significance between WT versus Pgam5 KO mice. How to cite this article : Lu, W. et al . Genetic deficiency of the mitochondrial protein PGAM5 causes a Parkinson’s-like movement disorder. Nat. Commun. 5:4930 doi: 10.1038/ncomms5930 (2014).